Local chiral symmetry breaking in triatic liquid crystals Understanding the behaviour of thermally excited many-particle systems, composed of a single particle type having a well-defined shape and size, is important in condensed matter, notably protein crystallization. Here we observe and explain the origin of local chiral symmetry breaking in a surprisingly simple system of hard Brownian particles: achiral regular triangles confined to two dimensions. Using enhanced optical video particle-tracking microscopy, we show that microscale lithographic triangular platelets form two different triatic liquid crystal phases. Above a particle area fraction φ A ≈0.55, the simple triatic phase is spatially disordered, yet has molecular orientational characteristics that distinguish it from a hexatic liquid crystal. At higher φ A ≥0.61, we find a second triatic phase exhibiting local chiral symmetry breaking; rotational entropy favours laterally offsetting the positions of nearest-neighbouring triangles. By contributing to spatial disordering, local chiral symmetry breaking can limit the range of shapes that can be entropically crystallized. The tendency of certain colloidal shapes to form ordered crystals [1] , [2] , [3] , [4] , [5] , [6] , even when subject to thermal excitations, is important in protein crystallization [1] , [7] and directed assembly [8] , [9] , [10] . Although some shapes readily crystallize, others do not [7] ; this limits the range of proteins structures that can be deduced by crystallography. Beyond crystallization, the most basic physical ingredients that can induce chiral symmetry breaking [11] , even locally, remain unclear [12] . Entropy-driven ordering in dense multi-particle systems can be strongly influenced by particle shape [9] , [13] , [14] , [15] , [16] , [17] , [18] , [19] , [20] . Although initially controversial, hard uniform spheres freeze through a spatial disorder–order transition as their number density is increased, yet well below the density at which the spheres pack and can no longer translate [3] , [4] , [21] . Such spatial ordering, which might seem paradoxical at first, provides greater translational free volume per sphere, thereby maximizing entropy. By contrast, the classic Onsager fluid, consisting of thin and long hard rods, undergoes a different type of phase transition, as the rod density is increased from a disordered isotropic (I) fluid phase, having short-range spatial and orientational order, to a nematic (N) liquid crystal phase, having short-range spatial order but long-range molecular-orientational (MO) order [15] . This I–N transition is driven by an increase in entropy: the loss of entropy suffered by the development of MO order is more than compensated by an increase in entropy due to a larger available translational free volume per rod. Thus, significant shape anisotropy can give rise to spatially disordered liquid crystal phases in multi-particle systems at high densities. The particular type of liquid crystal that forms can depend in a delicate way on a particle's precise shape and also on the dimensionality of space. For instance, in two dimensions (2D), as the density of hard discs is increased, the isotropic phase transforms into a classic hexatic (H) liquid crystal phase, which possesses quasi-long-range (QLR) six-fold bond-orientational (BO) order, yet only short-range spatial order [22] , [23] . In three dimensions (3D), differences in particle shapes give rise to a variety of liquid crystal phases, such as smectic [16] and discoidal phases [17] . Beyond classic liquid crystals [16] , new forms, such as the cubatic phase [9] , [24] , have been predicted but thus far not observed. Simulations of regular triangular prisms in 3D show a spatially ordered honeycomb crystal that simply melts into an isotropic phase without any intervening liquid crystal phase [9] ; some other complex polyhedra appear to form liquid crystal phases in 3D at high densities [9] . Among 2D shapes, the equilateral triangle is the simplest of all regular polygons, and its shape is inherently achiral. Nevertheless, the behaviour of dense Brownian systems of hard triangles has not been fully elucidated. An artificial neural network simulation of triangles in 2D (ref. 20 ) has predicted only a single type of high-density liquid crystal-like phase above a particle area fraction φ A ≈0.57, but its nature remains vague and mysterious. The advent of precisely controlled synthesis of dispersed colloidal systems, made by microlithography, has opened up new experimental realizations of many-body hard-core systems of precisely controlled shapes, having tailored anisotropic interactions [25] , [26] , [27] . In particular, roughness controlled depletion attractions [28] , [29] , a variation of shape-selective depletion attractions [30] , have yielded a route that enables experimental exploration of dense 2D systems of hard Brownian microscale platelets. These microscopic platelets are small enough that the thermal Brownian excitations at room temperature cause substantial fluctuations in positions and orientations of the particles, yet they are large enough that optical video microscopy can be used to visualize and record images of many particles in a single field of view. Studies of 2D systems of hard uniform pentagons [14] , which cannot fully tile a plane, have shown crystallization into a hexagonal rotator crystal (RX) phase that undergoes glassy-like rotational dynamic arrest and spatial disordering under higher compression. By contrast, 2D systems of hard squares [13] , which can fully tile a plane, exhibit a first-order crystal–crystal transition between a hexagonal rotator crystal and a rhombic crystal. The characteristic angle of the rhombic unit cell changes continuously towards a square phase under increasing compression. Although interesting and rich, the observed phases of squares and pentagons do not provide any clear predictive power for the phase behaviour of dense 2D systems of regular triangles. Using enhanced optical video particle-tracking microscopy, we study dense diffusing systems of hard regular triangular platelets confined to 2D by roughness-controlled depletion attractions [28] . In striking contrast to systems of squares and pentagons, we show the development of liquid crystal order from the isotropic phase, as φ A of the triangles is increased above φ A ≈0.55; corresponding Fourier transform intensities predominantly reveal the equilibrium structure factor. Spatial and orientational correlation functions, translational and rotational mean square displacements, and order parameters reveal the emergence of a simple triatic liquid crystal phase T Δ that reflects the underlying three-fold symmetry of the triangular particles. Vertices of triangles in the triatic phase effectively point along six well-defined directions in the plane over extended distances, and, around a given central triangle, the three nearest-neighbouring triangles point away from the central triangle. Beyond φ A ≈0.61, rotational entropy favours lateral offsetting of nearest-neighbouring triangles, yielding a triatic phase T Δχ that exhibits local chiral symmetry breaking (LCSB). Three sets of chiral enantiomeric building blocks, consisting of pairs of + and − offset dimers of triangles, can be equivalently used to analyse the real-space images, and over large distances compared with the triangle size, the T Δχ phase is racemic. Both in the T Δ and T Δχ phases, collective translational sliding motions of triangles along lubricated slip lines in the plane, defined by the orientational order, also have a role in the observed entropic fluctuations. Overall, the direct observation of LCSB in triatic liquid crystals of hard triangles shows that the simple combination of entropy and the geometric shape of the constituent particles is sufficient to induce chirality spontaneously, even if locally. Thus, LCSB can have an important role in limiting the range of shapes of colloidal objects, including proteins and other biological structures, that can be entropically crystallized. Structure of dense systems of hard Brownian triangles At φ A =0.52 ( Fig. 1a ), the rotationally symmetric ring pattern, in the structure factor, is indicative of liquid-like short-range spatial order. At higher φ A =0.56 ( Fig. 1b ), the liquid ring remains broadened, but the intensity has developed a six-fold azimuthal modulation in the Fourier transform. This modulation is reminiscent of the six-fold QLR-BO order of a hexatic liquid crystal [31] . We thus associate φ A ≈0.55 with a transition from an isotropic phase to a liquid crystal phase, as yet unclassified. At even higher φ A =0.58 ( Fig. 1c ), the modulations become more pronounced and extend to larger wavenumbers. For φ A ≥0.63 ( Fig. 1d ), six-fold MO order extends across the entire viewing region; triangles far from a chosen triangle have vertices that either point nearly in the same direction or in the opposite direction. The modulations are so pronounced at φ A =0.63 that they appear as six highly diffuse spots. At yet larger φ A =0.69 ( Fig. 1e ), these six spots around the primary ring are less diffuse and a second ring of six diffuse spots becomes better defined at higher wavenumbers, suggesting a greater degree of local spatial order ( Supplementary Fig. S1 ). 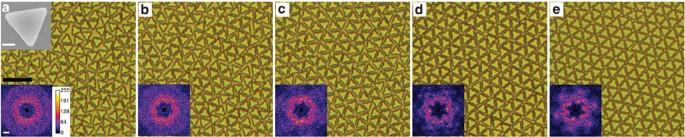Figure 1: Observed phases of hard regular triangular platelets. Optical microscope images of microscale triangular polymeric platelets, dispersed in aqueous solution, and confined by roughness-controlled depletion attractions to diffuse in a plane at particle area fractionsφA: (a) 0.52, (b) 0.56, (c) 0.58, (d) 0.63, and (e) 0.69. Scale bar for optical images, 10 μm. Insets in the lower left corners are Fourier transforms, where colours encode the intensities and scale bar is 0.2 μm−1. Inset in the upper left corner of partais a scanning electron micrograph of a triangular polymer platelet; scale bar, 1 μm. Figure 1: Observed phases of hard regular triangular platelets. Optical microscope images of microscale triangular polymeric platelets, dispersed in aqueous solution, and confined by roughness-controlled depletion attractions to diffuse in a plane at particle area fractions φ A : ( a ) 0.52, ( b ) 0.56, ( c ) 0.58, ( d ) 0.63, and ( e ) 0.69. Scale bar for optical images, 10 μm. Insets in the lower left corners are Fourier transforms, where colours encode the intensities and scale bar is 0.2 μm −1 . Inset in the upper left corner of part a is a scanning electron micrograph of a triangular polymer platelet; scale bar, 1 μm. Full size image Because the Fourier transform of an individual microscope image contains significant speckle, reflecting only a single configuration of triangles in a small viewing region at a particular instant (for example, see insets in Fig. 1 ), it is desirable to obtain a smoother average from different configurations of triangles, in a certain interrogation region, as the system fluctuates in equilibrium. From recorded movies, taken at different locations in the 2D column and therefore different φ A , we extract images every 3 s over a duration of 4.8 min, and then perform Fourier transforms for each extracted image. At each φ A , we obtain a time-averaged Fourier transform intensity pattern by summing all of the Fourier transform intensities, and then dividing the sum by the total number of Fourier transform images. Because the time-averaged Fourier transforms are six-fold symmetric, we also average over successively 60°-rotated versions, yielding smoother patterns. The results of these temporally and rotationally averaged Fourier transform intensity patterns for φ A =0.52, 0.58, 0.62 are shown in Fig. 2a–c , respectively. Comparing Fig. 2b with c , we find that features at higher wavenumbers are more intense and sharper for φ A =0.62 than for φ A =0.58. Light-scattering measurements of equilibrium 2D gravitational columns of triangles (Methods) also reveal a circularly symmetric intensity pattern for the lower-density isotropic phase and a six-fold symmetric intensity pattern of azimuthally smeared spots for higher φ A , as shown in Fig. 2d,e , respectively. 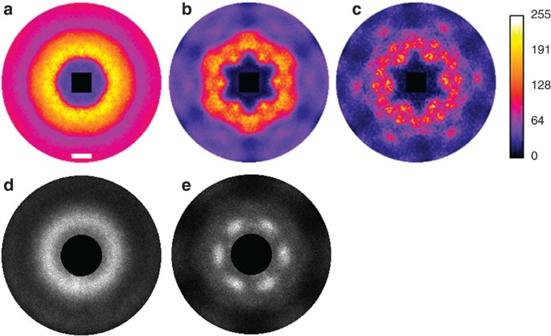Figure 2: Time-averaged Fourier transforms and light scattering. Reciprocal-space intensity patterns obtained from: time-averaging Fourier transforms of optical microscopy videos (a–c), and light-scattering measurements (d,e) of dense 2D systems of triangles. Fourier transform intensity patterns: (a) isotropic phase (φA=0.52); (b) TΔphase (φA=0.58); (c) TΔχphase (φA=0.62). Scale bar ina, 0.2 μm−1. Light-scattering intensity patterns: (d) dense isotropic phase; (e) average over high-density triatic phases. Fourier transform intensities ina–care encoded in colour (see colour scale bar on right). Central regions in all patterns at low wavenumbers have been removed for clarity (black squares and circles). Figure 2: Time-averaged Fourier transforms and light scattering. Reciprocal-space intensity patterns obtained from: time-averaging Fourier transforms of optical microscopy videos ( a – c ), and light-scattering measurements ( d , e ) of dense 2D systems of triangles. Fourier transform intensity patterns: ( a ) isotropic phase ( φ A =0.52); ( b ) T Δ phase ( φ A =0.58); ( c ) T Δχ phase ( φ A =0.62). Scale bar in a , 0.2 μm −1 . Light-scattering intensity patterns: ( d ) dense isotropic phase; ( e ) average over high-density triatic phases. Fourier transform intensities in a – c are encoded in colour (see colour scale bar on right). Central regions in all patterns at low wavenumbers have been removed for clarity (black squares and circles). Full size image Spatial and orientational correlation functions To classify liquid crystal phases precisely, it is necessary to calculate correlation functions: the spatial radial distribution function g ( r / D ), the three-fold MO correlation function g 3 mo ( r / D ), and the six-fold MO correlation function g 6 mo ( r / D ), where r is the centre-to-centre distance between two triangles and D is the diameter of a circle circumscribed around a triangle (Methods). Using trajectories of particles obtained by optical video particle-tracking microscopy (see Methods and Supplementary Fig. S2 ), we find that g ( r / D ) rapidly decays to a limiting value of unity at large r beyond a few D ( Fig. 3a ), so there is no QLR spatial order even at the highest φ A we observe. Next, g 3 mo ( r / D ) shows a striking negative short-range anti-correlation peak of −1 at small r / D ( Fig. 3b ). Remnants of this peak are discernible even for φ A as low as ≈0.35, indicating local antiparallel orientation of at least some nearest-neighbouring triangles. However, for larger r / D , g 3 mo also rapidly approaches its asymptotic value of zero, so there is no three-fold QLR–MO order at any φ A we observe. By contrast, g 6 mo ( r / D ), does exhibit six-fold QLR–MO order at larger φ A ( Fig. 3c ): at φ A =0.42, g 6 mo ( r / D ) decays rapidly, at φ A =0.52, the decay in g 6 mo is slower but still approaches zero towards large r / D , and for higher φ A , g 6 mo decays relatively little over the range of r / D in a single image. Thus, above φ A ≈0.55, we identify a new thermodynamic liquid crystal phase, which has six-fold QLR–MO order, yet local anti-correlation in the three-fold MO order, as a simple triatic liquid crystal phase: T Δ . 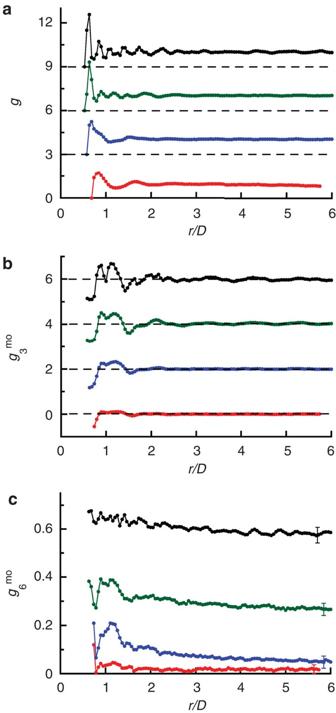Figure 3: Spatial and orientational correlation functions. (a) Spatial pair correlation functiong. (b) Three-fold molecular orientational correlation functiong3mo. (c) Six-fold molecular orientational correlation functiong6mo. Hereris the centre-to-centre separation between triangles,D=(2/31/2)Lis the diameter of a circumscribed circle around a triangle, andLis the average edge length of a triangle. Triangle area fractions in each panel are:φA=0.64 (black), 0.58 (green), 0.52 (blue), and 0.42 (red). Inaandb, the traces are offset for clarity; horizontal dashed lines show zero levels for corresponding correlation functions; error bars incare s.d. Figure 3: Spatial and orientational correlation functions. ( a ) Spatial pair correlation function g . ( b ) Three-fold molecular orientational correlation function g 3 mo . ( c ) Six-fold molecular orientational correlation function g 6 mo . Here r is the centre-to-centre separation between triangles, D =(2/3 1/2 ) L is the diameter of a circumscribed circle around a triangle, and L is the average edge length of a triangle. Triangle area fractions in each panel are: φ A =0.64 (black), 0.58 (green), 0.52 (blue), and 0.42 (red). In a and b , the traces are offset for clarity; horizontal dashed lines show zero levels for corresponding correlation functions; error bars in c are s.d. Full size image Rotational and translational dynamics The identification of different phases is also evident from changes in the rotational and translational dynamics of individual triangles. The ensemble-averaged time-dependent mean square angular displacement (MSAD) 〈Δ θ 2 ( t )〉 and the 2D mean square displacement (MSD) 〈Δ r 2 ( t )〉 for individual triangles are shown for a series of φ A in Fig. 4 . The ensemble size used for averaging is ≈250 triangles, and the time duration is about 5 min. At φ A =0.42 and 0.52, the MSADs are sub-diffusive at early times and become diffusive at longer times ( Fig. 4a ). By contrast, for higher φ A ≥0.58, the MSADs exhibit plateaus that decrease in magnitude; a long-time plateau indicates a transition from rotational ergodicity to non-ergodicity and is correlated with the onset of QLR–MO order. Individual triangles are no longer able to rotate and explore all possible orientations because of cage-like confinement by neighbouring triangles (see, for example, Fig. 1b–e ). This caged rotational diffusion of triangles additionally differentiates T Δ from the classic H phase of discs, which exhibit unbounded rotational diffusion since they are not packed into frictional contact. 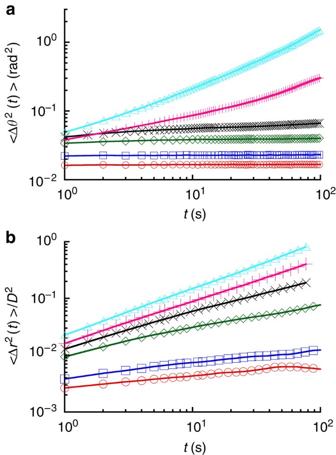Figure 4: Time- and ensemble-averaged mean square displacements. (a) MSADs 〈Δθ2(t)〉; (b) normalized two-dimensional translational MSDs 〈Δr2(t)〉/D2, whereDis a circumscribed circle's diameter andtis time, at particle area fractionsφA=0.42 (aqua), 0.52 (pink), 0.58 (black), 0.61 (green), 0.63 (blue), and 0.64 (red). Lines guide the eye. Figure 4: Time- and ensemble-averaged mean square displacements. ( a ) MSADs 〈Δ θ 2 ( t )〉; ( b ) normalized two-dimensional translational MSDs 〈Δ r 2 ( t )〉/ D 2 , where D is a circumscribed circle's diameter and t is time, at particle area fractions φ A =0.42 (aqua), 0.52 (pink), 0.58 (black), 0.61 (green), 0.63 (blue), and 0.64 (red). Lines guide the eye. Full size image Interestingly, the ensemble-averaged translational dynamics are quite different than the rotational dynamics. At low φ A =0.42, the MSD is diffusive at long times, whereas it becomes gradually more and more sub-diffusive as the density increases towards φ A =0.64 ( Fig. 4b ). Even though individual triangles are heavily constrained by a cage of neighbours for larger φ A , this does not necessarily imply that there are no strong positional thermal fluctuations because of the possibility of collective transport. Careful inspection of the videos at higher φ A shows that there indeed exist significant sliding fluctuations of many triangles via collective motion along six different slip directions that are dictated by the six-fold QLR–MO order ( Supplementary Movies 1 and 2 ). Thermal fluctuations can drive collective translational motion of many triangles in concert without significantly disturbing their orientations at essentially no cost in energy, indicating a significant translational sliding degeneracy. Real-space observation of local chiral symmetry breaking For φ A well above the I–T Δ transition, we observe that the edges of the three nearest-neighbouring triangles are often misaligned with the edges of a given central triangle. We calculate the probability distribution p ( d sh / D ) of a first nearest-neighbouring antiparallel triangle that is shifted by a transverse displacement d sh , relative to a given test triangle ( Fig. 5a ). A symmetric monomodal peak centred around d sh / D =0 is found for φ A <0.6. In this regime, nearest-neighbouring triangles are, on average, aligned with a central test triangle, yet, there are a significant number of nearest-neighbouring triangles that have plus-and-minus lateral offsets (that is, transverse shifts) with equal probabilities; we choose counterclockwise shifting to be positive. However, for φ A ≥0.61, we clearly resolve a symmetric double peak in p ( d sh / D ), indicating a preferred magnitude for a transverse offset, producing two dominant, distinct and equal populations of left- and right-shifted dimers of triangles. This quantitatively demonstrates that entropy alone can induce LCSB in a dense system of achiral particles [11] , [12] . 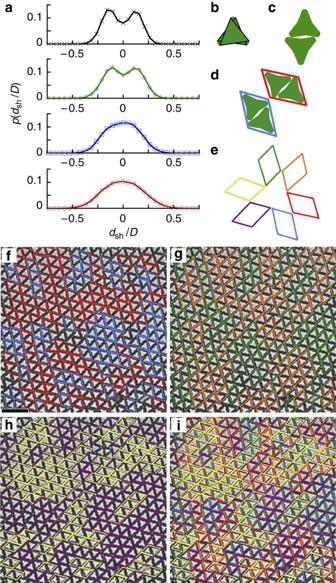Figure 5: Triatic phase revealing LCSB. A high-density triatic liquid crystalline phase TΔχof hard triangles exhibits LCSB: (a) probability distributions of finding a first nearest-neighbouring triangle having a lateral normalized offsetdsh/Dfor particle area fractionsφA=0.52 (red), 0.58 (blue), 0.61 (green), and 0.63 (black). A racemic mixture of offset dimers emerges as the most probable local configuration forφA>0.6, as evidenced by the double peak, reflecting the importance of rotational entropy. (b) A triangle is rotated about its centre over a limited angle, and the trioid shape (green region) is defined as the total area that the triangle sweeps out during the rotation (black outlines show the triangle at initial and final orientations). (c) A pair of trioids pack more efficiently when offset, forming the motif of an offset dimer of triangles. (d) Lateral offsets of triangles can be along either + or − direction, yielding a pair of offset dimers (enclosed by red and blue parallelograms) as a basis set for analysis. (e) Pairs of parallelograms can be used to enclose + shifted and − shifted offset dimers of triangles. Three different equivalent basis pairs of offset dimers (parallelograms: red and blue, green and orange, purple and yellow, respectively). (f–i) Dimer basis analysis of triangles atφA=0.69 using the following offset pairs: (f) red/blue, (g) green/orange, (h) purple/yellow, and (i) composite of all three basis sets overlayed, showing equivalence of coverage. Scale bar inf, 10 μm. Figure 5: Triatic phase revealing LCSB. A high-density triatic liquid crystalline phase T Δχ of hard triangles exhibits LCSB: ( a ) probability distributions of finding a first nearest-neighbouring triangle having a lateral normalized offset d sh / D for particle area fractions φ A =0.52 (red), 0.58 (blue), 0.61 (green), and 0.63 (black). A racemic mixture of offset dimers emerges as the most probable local configuration for φ A >0.6, as evidenced by the double peak, reflecting the importance of rotational entropy. ( b ) A triangle is rotated about its centre over a limited angle, and the trioid shape (green region) is defined as the total area that the triangle sweeps out during the rotation (black outlines show the triangle at initial and final orientations). ( c ) A pair of trioids pack more efficiently when offset, forming the motif of an offset dimer of triangles. ( d ) Lateral offsets of triangles can be along either + or − direction, yielding a pair of offset dimers (enclosed by red and blue parallelograms) as a basis set for analysis. ( e ) Pairs of parallelograms can be used to enclose + shifted and − shifted offset dimers of triangles. Three different equivalent basis pairs of offset dimers (parallelograms: red and blue, green and orange, purple and yellow, respectively). ( f – i ) Dimer basis analysis of triangles at φ A =0.69 using the following offset pairs: ( f ) red/blue, ( g ) green/orange, ( h ) purple/yellow, and ( i ) composite of all three basis sets overlayed, showing equivalence of coverage. Scale bar in f , 10 μm. Full size image The origin of LCSB in dense Brownian systems of hard triangles can be understood by effectively incorporating the effect of rotational entropy into a new particle shape based on a triangle. Consider a rotationally swept triangle that is rotated back and forth symmetrically about its centre over a specific range of angles Δ θ , generating a trioid shape ( Fig. 5b ). This trioid shape effectively captures the range of orientations of triangles that are caged by neighbouring triangles at high φ A . Two equivalent local packing arrangements of a pair of trioids maximize Δ θ and thus the rotational entropy: two nearest-neighbouring antiparallel trioids are shifted to form either of two chiral isomers (that is, + or −) of the offset dimer motif ( Fig. 5c ). To graphically show the racemic mixture of offset dimers at high φ A , we consider only the two average configurations corresponding to the double-peak in the probability distribution p ( d sh / D ), which determine two parallelogram-shaped isomers that enclose corresponding pairs of dimers ( Fig. 5d ). Since each of the six different directions in the plane, defined by the QLR–MO order, is associated with a parallelogram, three sets of two parallelograms (that is, pairs of + and − offset dimers) can be equivalently used as a basis for analysis ( Fig. 5e ). The average sizes of the regions having a similar sense of parallelogram define a correlation length for the LCSB, which is typically about 4–5 particle diameters, yet the entire system remains racemic at large length scales ( Fig. 5f–i ). Although parallelograms can be used to analyse nearly all triangles in a given image, we also observe some defects, such as dislocations and disclinations. Among these, head-tail local configurations create frustration and lie outside the offset dimer analysis scheme. The inter-related changes in the measured structural and dynamic characteristics of the hard triangle system are summarized in Fig. 6 . The increase in the average antiparallel nature of nearest-neighbouring triangles is seen in the three-fold local MO average 〈cos(3 δθ )〉, where δθ represents the relative angle between a given test triangle and its first nearest neighbour ( Fig. 6a ). At low φ A <0.35, the MO is isotropic, so 〈cos(3 δθ )〉 ∼ 0. For φ A >0.35 (near the limit 0.375 of circumscribed triangles packed in 2D, φ A *= φ hd ( A tri / A disc )=[ π /(12) 1/2 ][3 3/2 /(4 π )]=3/8, where φ hd is the area fraction of hexagonally packed discs in a plane, and A tri / A disc is the area fraction of a triangle inside its circumscribed circle (inset, Fig. 6a )), we observe a gradual decrease in 〈cos(3 δθ )〉 towards complete antiparallel correlation (that is, −1). Simultaneously, the short-range local anti-correlation peak in g 3 mo rises, indicating that local edge–edge configurations of triangles become more prevalent than edge–tip or tip–tip configurations as φ A increases. φ A * would be a lower-bound on the onset area fraction associated with a hypothetically possible RX phase of triangles. However, although there is a gradual increase in the MO anisotropy of nearest-neighbouring triangles above φ A *, we do not observe a RX phase for triangles. Instead, triangles have a high-enough effective aspect ratio to suppress the RX phase compared with other regular polygons such as squares [13] and pentagons [14] , which do have RX phases. Of all regular polygons, triangles have the highest effective aspect ratio, defined as the centre-to-vertex distance divided by the centre-to-nearest-edge distance, equal to 2. This aspect ratio is high enough to enable the formation of a molecularly oriented liquid crystal phase. 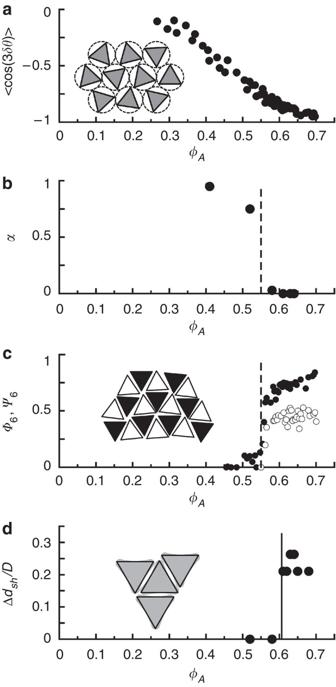Figure 6: Dependence of order parameters on particle area fraction . (a) Average degree of antiparallel alignment, given by 〈cos(3δθ)〉, of first nearest-neighbouring triangles having centre-to-centre separationsr≤(3/4)D, where 〈cos(3δθ)〉=−1 corresponds to perfectly antiparallel molecular orientations of the first nearest-neighbouring triangle (inset:φA*=0.375 for triangles corresponding to 2D hexagonal packing of circles that circumscribe them). (b) Power law exponentαof the MSAD in the long-time limit 〈Δθ2(t)〉∼tα. (c) Six-fold MO order parameterΦ6(solid circles) and hexatic six-fold BO order parameter of next nearest neighboursΨ6(open circles): inset shows interpenetrating lattices of up and down triangles; dashed vertical lines forbandcatφA≈0.55 indicate a transition to a triatic liquid crystal phase TΔhaving quasi-long-range MO and BO order. (d) Normalized separation Δdsh/Dbetween the double peak inp(dsh/D) provides a measure of LCSB that yields stereo-isomers of dimers of triangles having +/− lateral offsets: inset shows an example of a central triangle having three nearest-neighbouring triangles (light-grey shadows show trioid constructions, one nearest-neighbouring triangle has − lateral offset (clockwise) and two nearest-neighbouring triangles have + lateral offsets (counter-clockwise)). Vertical solid line indicates a transition aroundφA≈0.61 to a higher density TΔχphase exhibiting LCSB. Figure 6: Dependence of order parameters on particle area fraction . ( a ) Average degree of antiparallel alignment, given by 〈cos(3 δθ )〉, of first nearest-neighbouring triangles having centre-to-centre separations r ≤(3/4) D , where 〈cos(3 δθ )〉=−1 corresponds to perfectly antiparallel molecular orientations of the first nearest-neighbouring triangle (inset: φ A * =0.375 for triangles corresponding to 2D hexagonal packing of circles that circumscribe them). ( b ) Power law exponent α of the MSAD in the long-time limit 〈Δ θ 2 ( t )〉 ∼ t α . ( c ) Six-fold MO order parameter Φ 6 (solid circles) and hexatic six-fold BO order parameter of next nearest neighbours Ψ 6 (open circles): inset shows interpenetrating lattices of up and down triangles; dashed vertical lines for b and c at φ A ≈0.55 indicate a transition to a triatic liquid crystal phase T Δ having quasi-long-range MO and BO order. ( d ) Normalized separation Δ d sh / D between the double peak in p ( d sh / D ) provides a measure of LCSB that yields stereo-isomers of dimers of triangles having +/− lateral offsets: inset shows an example of a central triangle having three nearest-neighbouring triangles (light-grey shadows show trioid constructions, one nearest-neighbouring triangle has − lateral offset (clockwise) and two nearest-neighbouring triangles have + lateral offsets (counter-clockwise)). Vertical solid line indicates a transition around φ A ≈0.61 to a higher density T Δχ phase exhibiting LCSB. Full size image By contrast, the system's rotational dynamics and orientational order change abruptly at the I–T Δ transition. The power law exponent α , characterizing the rotational diffusion at long times 〈Δ θ 2 ( t )〉 ∼ t α , drops dramatically at ( Fig. 6b ), indicating strongly caged rotational diffusion of triangles above (dashed line, Fig. 6b ). Structurally, we find a rapid increase in the six-fold MO order parameter Φ 6 and in the hexatic six-fold BO order parameter for next-nearest-neighbouring triangles Ψ 6 ( Fig. 6c ) (see also Methods and Supplementary Fig. S3 ). The sharp changes in α , Φ 6 , and Ψ 6 at indicate that dynamics and structure are closely linked through the I–T Δ transition. To quantify the onset of LCSB, we calculate Δ d sh / D , which describes the total lateral shift between the two peaks in the probability distribution p ( d sh / D ) ( Fig. 6d ). This dimensionless parameter is zero below about φ A ∼ 0.61, because there is only one peak in p , and it rises abruptly to a value near Δ d sh / D ≈0.25, for larger 0.61< φ A ≤0.7. Thus, φ A ≈0.61 is the transition between simple T Δ having a single peak in p ( d sh / D ) and the LCSB triatic phase T Δχ , which possesses a clearly resolved double peak in p ( d sh / D ). The lateral offsets associated with LCSB reduce Ψ 6 , so it only rises to a value of about 0.5 ( Fig. 6c ). Additionally, the collective translational sliding degeneracies of the triangles further reduce Ψ 6 without affecting Φ 6 to nearly the same degree. The trioid model predicts that Δ d sh ( φ A )/ D will decrease towards zero at very high compression. In the T Δχ phase, the chiral symmetry is only broken locally: the system as a whole is a racemic mixture of small chiral domains. The double-peak in p is associated with the formation of offset dimer triangle-pairs having two stereo-isomer variants in equal proportions; thus, LCSB effectively results from maximizing the combined rotational and translational entropy. Moreover, the local chiral asymmetry, which is racemic, never becomes long-range of a single enantiomer type, even as thermal fluctuations can continuously drive changes in the signs of local offsets. Collective translational sliding fluctuations along slip lines also aids in the destruction of spatial order, even as orientational fluctuations become strongly quenched. The observation of entropy-driven LCSB, in 2D liquid crystals of hard regular triangles, is remarkable, especially because other regular polygons that have smaller aspect ratios, such as squares and pentagons [13] , [14] , do not exhibit LCSB. The combination of LCSB and collective translational sliding in triatic liquid crystals, despite the symmetry and monodispersity of achiral triangular constituents, can thus act to frustrate entropic spatial crystallization. Because LCSB can contribute to spatial disordering, it can limit the range of shapes, even if highly symmetric, that can be entropically crystallized. Indeed, we anticipate that rotational entropy of sufficiently anisotropic hard particles could also lead to LCSB in dense 3D systems. The emergence of two types of triatic liquid crystal phases, including one that exhibits LCSB, indicates that the subtle combination of geometry and entropy may combine to produce yet further surprises for other shapes, whether in two or three dimensions. 2D osmotic compression and measurement of area fraction Equilateral triangular platelets (that is, triangles) having edge length L =3.7±0.1 μm and thickness h =2.0±0.1 μm are fabricated from SU-8 polymer by photolithography, released into aqueous solution, and stabilized against aggregation by adsorbed sodium dodecyl sulfate (1 mM). We mix a dilute dispersion of triangles ( ∼ 5×10 −4 v/v) with a dispersion of nanoscale polystyrene spheres, which act as a depletion agent, and seal the mixture in a rectangular glass microcapillary (0.2 mm×4.0 mm×20 mm). The size and concentration of polystyrene spheres (polystyrene spheres: diameter ∼ 0.02 μm, concentration ∼ 0.5% w/v, sulfate-stabilized) are selected to cause desired anisotropic attractions that leads to a good realization of a 2D hard-core system: roughness-controlled depletion attractions between the faces of the triangles and the microcapillary surface are strong enough, relative to thermal energy to inhibit Brownian rotational or translational excitations out of the plane [28] , yet the triangles retain their capacity to diffuse translationally and rotationally in the plane. The triangles are osmotically compressed by gravity in the plane by slightly tilting the microcapillary, between about 2° and 5°, with respect to the horizontal. Because the particles have a higher mass density ( ρ SU8 ≈1.2 g cm −3 ) than water, the 2D osmotic pressure Π at a given location in the monolayer arises from the effective gravitational mass of particles above it, projected along the tilted plane. The system achieves a steady state after several weeks, when the concentration profile as a function of distance along the microcapillary stops changing, as measured using optical video microscopy (Nikon Eclipse TE2000 inverted microscope, ×40 plan-apo long working distance objective lens with correction collar, brightfield transmission illumination; Point Grey Flea2 colour CCD camera, 8-bit depth per colour channel, 1,024×768 pixels, 30 Hz max acquisition rate). In this steady-state 2D column of particles, Π increases towards the lower regions of the monolayer, so the particle area fraction φ A also increases, yielding a slowly varying gradient in φ A within the monolayer. About 400 particles can be observed in a single field of view (64 μm×64 μm) at high φ A . All φ A are calculated using particle centre locations, determined by tracking software, and the average measured size of the triangles, determined by scanning electron microscopy. Because of edge roughness of the triangles, effective area fractions may be slightly larger (for example, 1–2%) than our reported values. In 2D colloidal systems of microscopic particles, the particle area fraction φ A corresponds directly to the particle density associated with phase transitions, whereas, in condensed molecular systems (which have significant intermolecular attractions, not just hard-core repulsions), altering the temperature is often used to change the molecular density in addition to the degree of thermal fluctuations. Enhanced particle-tracking image analysis We have created enhanced video particle-tracking microscopy software, improving on existing routines for isotropic spheres and discs (for example, refs 32 , 33 ), by detecting not only the centre position but also a vertex of every triangle in each successive video frame, thereby providing both positional and orientational trajectories as a function of time ( Supplementary Fig. S2 ). These measured particle trajectories are then used to calculate ensemble-averaged spatial, orientational and dynamical correlation functions, order parameters, and mean square displacements. Fourier transforms of video images For each image, using standard procedures, we crop a 512 pixel×512 pixel portion of the image from the centre of the raw 550 pixel×550 pixel image, convert to grayscale, and use the standard fast Fourier transform command in Interactive data language software to perform the Fourier transform. This command returns a 512 pixel×512 pixel grayscale Fourier transform intensity having 8-bit dynamic range. Because the primary features of interest in the Fourier transform are within a 100 pixel×100 pixel region at the centre, we crop the Fourier transform and only show this smaller region. We block the centre of the Fourier transform using a small black square (7 pixel×7 pixel). We use a colour look-up table to colour-code the intensity values over the range from zero to 255. By making separate image files of dots at the centre positions of the triangles and taking the Fourier transform ( Supplementary Fig. S1 ), we have verified that the Fourier transform patterns of the microscope images, shown in the insets of Fig. 1a , dominantly reflect the triangles' positional structure, that is, centre-to-centre locations of triangles and structure factor S ( q ), where q is the wavevector, rather than the form factor F ( q ) of a single-triangle shape. The six-fold intensity modulation of S ( q ) can be effectively attributed to BO order. In dense systems of triangles, BO order is inherently coupled to MO order. So besides g 6 mo , the six-fold BO correlation function g 6 bo for next nearest-neighbouring triangles also shows the developing of QLR order as φ A increases ( Supplementary Fig. S3 ). Light-scattering measurements A helium–neon laser beam (Melles Griot, wavelength 632.8 nm, beam waist 650 μm, power 15 mW) illuminates the monolayer of triangles. The scattering pattern is formed on a screen located 10 cm beyond the sample and recorded by a monochrome CCD camera (Point Grey: Flea). The light-scattering patterns in Fig. 2d,e are smoother than the averaged Fourier transforms, which is expected when averaging over a much larger number of triangles in the illuminated region (as compared with the microscope images). However, because there is a gradient in φ A in the column, and the illuminating beam waist is much larger than the viewing region in the microscope, these light-scattering patterns represent averages over relatively large ranges of φ A . We have made an attempt to obtain light-scattering patterns at well-defined φ A by reducing the beam waist (for example, to illuminate about the number of particles, as in our microscope images); however, this reduction in illumination area makes the light-scattering intensity patterns significantly less smooth and speckled, so they essentially resemble what we obtain from Fourier transform of individual microscope images. To obtain superior intensity patterns in reciprocal space at a single well-defined φ A , it would be desirable to perform light scattering by illuminating an extended area of a uniform 2D system of triangles, if an alternative method for concentrating the particles, which does not create a gradient in φ A , could be developed. Order parameters and correlation functions General definitions of order parameters and correlation functions have been published previously (see ref. 13 ). In particular, for triangular shapes, the global m -fold molecular orientational order parameter Φ m is: where θ j is the orientation angle of particle j and N is the total number of particles. To remove the degeneracy of molecular orientation due to the three-fold symmetry of triangles, we use How to cite this article: Zhao, K. et al . Local chiral symmetry breaking in triatic liquid crystals. Nat. Commun. 3:801 doi: 10.1038/ncomms1803 (2012).